Global-scale latitudinal patterns of plant fine-root nitrogen and phosphorus Most water and essential soil nutrient uptake is carried out by fine roots in plants. It is therefore important to understand the global geographic patterns of fine-root nitrogen and phosphorus cycling. Here, by compiling plant root data from 211 studies in 51 countries, we show that live fine roots have low nitrogen (N) and phosphorus (P), but similar N:P ratios when compared with green leaves. The fine-root N:P ratio differs between biomes and declines exponentially with latitude in roots of all diameter classes. This is in contrast to previous reports of a linear latitudinal decline in green leaf N:P, but consistent with nonlinear declines in leaf litter N:P. Whereas the latitudinal N:P decline in both roots and leaves reflects collective influences of climate, soil age and weathering, differences in the shape of the response function may be a result of their different N and P use strategies. As the below-ground analogue of leaves for resource uptake, fine roots are responsible for water and nearly all essential soil nutrient uptake by plants. The global N pool in fine roots is estimated to be 4.8×10 8 Mg, approximately 1/7 of all terrestrial vegetation [1] . Nutrient release from decomposing roots is a key pathway of significant nutrient flux in terrestrial ecosystems [2] . In forests, for example, the amount of nutrients cycled to the soil via fine-root production and decomposition may equal to or even exceed those of above-ground litterfall [3] . Given the importance of fine-root carbon (C), N and P chemistry in biology, physiology, biogeochemistry,and plant-insect and plant-disease interactions [4] , it is important to understand geographic patterns in root N and P at a global scale and possible links to ecosystem-scale biogeochemical cycling. Ecological stoichiometry, in particular N:P ratios in plant green leaves, has been used to infer potential nutrient limitation of net primary production [5] and plant-herbivore interactions in food webs [4] . So far, terrestrial ecologists and physiologists have largely focused on ratios of N:P in plant green leaves [6] , [7] , but also somewhat on senesced-leaf litter [8] , [9] . By contrast, our understanding of N and P stoichiometry in root systems, especially at a global scale, is much less developed. Plant N and P stoichiometry is related to the variation among species, plant developmental stages, tissue types and environments [6] , [9] , [10] , [11] , [12] . Plant green-leaf N and P concentrations have been shown to vary among climatic and soil environments, presumably reflecting both plant adjustment (acclimation and adaptation) [13] and biogeographical differences in relative N and P supply [14] . Studies on both plant leaves [6] , [7] , [8] , [15] and on litterfall [8] , [9] indicate that broad latitudinal and biome-level differences in soil N and P supplies can result in differences in plant nutrition and ecosystem nutrient cycles. As metabolically active tissues, fine roots, similar to green leaves, might be expected to have similar N-to-P stoichiometry [7] at local and global scales. However, fine roots differ profoundly from green leaves in many other ways in terms of morphology, chemistry and metabolism [16] , and as a result could differ from leaves in N and P concentrations and ratios. For example, the requirement for N in Rubisco leads to a greater N concentration per unit C lost in dark respiration for leaves than roots [17] and could also lead to green leaves requiring more N relative to P than fine roots, which would result in differences in N to P stoichiometry between these two types of tissues. Given that the soil total N is often lower in both very young and very old soils than in middle-aged soils [18] , [19] and that soil age generally decreases with latitude [14] , [20] , N concentration in fine roots is expected, in a similar manner to that in leaves [6] , [9] , [10] , to increase, peak, and then decrease with increasing latitude. However, some studies have found that the extent of soil N limitation is not associated with latitude [21] , indicating that N concentration in fine roots may not change with latitude. By contrast, fine-root P is expected to decrease (and N:P ratio to increase) with decreasing latitude because of low soil P availability in low latitudes due to geologically older and highly leached P-limited soils [11] , [14] . Also, as stated in the latitudinal compensation hypothesis, species or populations from high-latitude environments may enhance their basal metabolic rates and have high potential growth rates to compensate for the short period of growing seasons [22] , [23] , [24] . Therefore, plant tissues such as leaves and fine roots of fast-growing species at high latitudes, based on the growth rate hypothesis [25] , are expected to have high P demand for P used in P-rich RNA in ribosomes that are needed for synthesis of proteins, thus leading to low N:P ratio at high latitudes. However, at present, we do not know whether global-scale plant fine-root latitudinal patterns are similar to the linear decline in N:P in green leaves [6] or to the nonlinear decline in N:P in senesced-leaf litter [8] . Here we compile data from 211 published studies on plant roots and show that the N:P ratio in roots declines exponentially with latitude in contrast to a linear decline in green leaves. Differences in root N:P ratios were largely due to variation in root P and were associated with variation in soil P rather than soil N, supporting the hypothesis that global latitudinal patterns of plant N:P are driven largely by soil P, providing support for the latitudinal compensation hypothesis and the growth rate hypothesis. 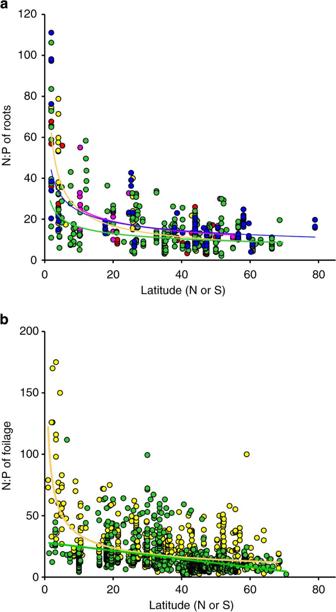Figure 1: N to P ratios in relation to latitude. (a) Root N:P ratios are best described by the power regressions (Φ<1 mm:y=55.7×latitude−0.366,r2=0.379,n=111, blue circles with blue trend line; 1≤Φ<2 mm:y=34.1×latitude−0.324,r2=0.188,n=374, green circles with green trend line; 2≤Φ<5 mm:y=56.6×latitude−0.463,r2=0.484,n=74, red circles with red trend line; Φ≥5 mm:y=90.1×latitude−0.562,r2=0.575,n=47, yellow circles with yellow trend line; and dead roots:y=66.6×latitude−0.420,r2=0.305,n=34, pink circles with pink trend line) and (b) green-leaf N:P ratio (data from references6,8) is best described by a linear function (y=28.2–0.334×latitude,r2=0.174,n=903, green circles with green trend line), and senesced-leaf N:P ratio (data from references8,9) is best described by a power function (y=122.3×latitude−0.547,r2=0.284,n=636, yellow circles with yellow trend line), all relationships are significant atP<0.0001. Root nutrients and their ratios in relation to root size We found that C concentration generally increased modestly, and N and P concentrations decreased with root size ( Table 1 ). N:P ratios tended to be higher in coarse roots >5 mm in diameter than in roots of <1, 1≤Φ<2, 2≤Φ<5 mm classes, which did not differ from each other, whereas C:N and C:P increased with root size in live roots ( Table 1 ). Compared with live roots of similar sizes, dead roots had generally lower C and P concentrations, but similar N concentrations. Thus, dead roots had higher N:P than live roots, but the patterns of C:N and C:P are inconsistent due to limited sample sizes ( Table 1 ). The lower P concentrations in dead than live roots (especially given no parallel pattern for N), may indicate P resorption from roots prior to senescence. Table 1 Root nutrients and their ratios in relation to root size at the global scale. Full size table Latitudinal patterns of root nutrients and their ratios There were significant relations of root N:P ratios to latitude ( Fig. 1 ). The N:P ratio both in live roots of all diameter classes and dead roots showed exponential declines with latitude ( r 2 for live roots <1 mm, 1≤Φ<2 mm, 2≤Φ<5 mm and ≥5 mm in diameter are 0.38, 0.19, 0.48 and 0.58, respectively; r 2 for dead roots is 0.31) ( Fig. 1a ). The exponential declines of root N:P ratios with latitude were similar to that of senesced leaves ( r 2 =0.284), but they differed from the linear and weaker decline in green leaves ( r 2 =0.174) ( Fig. 1b ). Figure 1: N to P ratios in relation to latitude. ( a ) Root N:P ratios are best described by the power regressions (Φ<1 mm: y =55.7×latitude −0.366 , r 2 =0.379, n= 111, blue circles with blue trend line; 1≤Φ<2 mm: y =34.1×latitude −0.324 , r 2 =0.188, n= 374, green circles with green trend line; 2≤Φ<5 mm: y =56.6×latitude −0.463 , r 2 =0.484, n= 74, red circles with red trend line; Φ≥5 mm: y =90.1×latitude −0.562 , r 2 =0.575, n= 47, yellow circles with yellow trend line; and dead roots: y =66.6×latitude −0.420 , r 2 =0.305, n= 34, pink circles with pink trend line) and ( b ) green-leaf N:P ratio (data from references [6] , [8] ) is best described by a linear function ( y =28.2–0.334×latitude, r 2 =0.174, n= 903, green circles with green trend line), and senesced-leaf N:P ratio (data from references [8] , [9] ) is best described by a power function ( y =122.3×latitude −0.547 , r 2 =0.284, n= 636, yellow circles with yellow trend line), all relationships are significant at P <0.0001. Full size image For fine roots, N, P and N:P ratio differed significantly among biomes ( Fig. 2 ). Among ecosystem types that had a sufficient number of observations ( n ≥25), the mean N in fine roots varied but did not show a consistent pattern in relation to the temperature and precipitation gradients ( Fig. 2a ), whereas the mean P increased in an order of tropical forests < tropical grasslands < temperate forests < temperate grasslands≈boreal forests ( Fig. 2b ). As a consequence, the mean N:P ratio decreased in the same order ( Fig. 2c ), which is consistent with the latitudinal pattern observed in Fig. 1 . 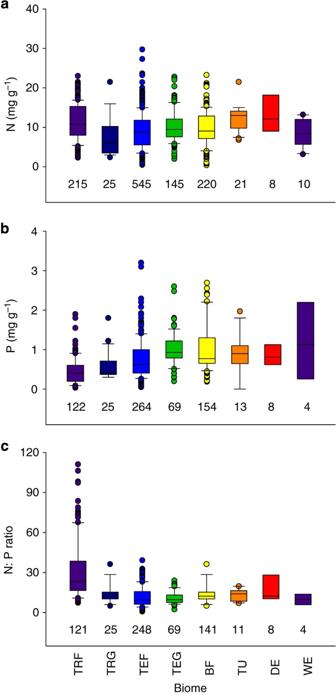Figure 2: Fine-root N and P stoichiometry among ecosystem types. (a) Fine-root N concentration, (b) Fine-root P concentration, (c) Fine-root N:P ratio. One-way analysis of variance is used to test the differences among BF, TEF, TRF, TEG, TRG, TU, deserts (DE) and wetlands (WE). The numbers in the figures are sample sizes for respective ecosystem types. The box plots summarize the distribution of points for each variable and group. The central box in each box plot shows the inter-quartile range, median (horizontal line in the box), 10th and 90th percentiles (lower and upper error bars) and individuals in the lower 10th percentiles (solid circles) for each group. BF, boreal forests; TEF, temperate forests; TEG, temperate grasslands; TRF, tropical forest; TRG, tropical grasslands; TU, tundra. Figure 2: Fine-root N and P stoichiometry among ecosystem types. ( a ) Fine-root N concentration, ( b ) Fine-root P concentration, ( c ) Fine-root N:P ratio. One-way analysis of variance is used to test the differences among BF, TEF, TRF, TEG, TRG, TU, deserts (DE) and wetlands (WE). The numbers in the figures are sample sizes for respective ecosystem types. The box plots summarize the distribution of points for each variable and group. The central box in each box plot shows the inter-quartile range, median (horizontal line in the box), 10th and 90th percentiles (lower and upper error bars) and individuals in the lower 10th percentiles (solid circles) for each group. BF, boreal forests; TEF, temperate forests; TEG, temperate grasslands; TRF, tropical forest; TRG, tropical grasslands; TU, tundra. Full size image Both climatic variables (mean annual temperature, MAT and mean annual precipitation, MAP), and soil variables (total soil N and P contents) were significantly associated with fine-root C, N, P and their ratios ( Table 2 ). For all fine-root (<2 mm in diameter) data pooled, N did not vary with MAT, but fine-root P decreased ( r 2 =0.203) with MAT. Fine-root N increased (albeit very weakly) and fine-root P decreased with MAP. Fine-root P decreased and N:P ratio increased, respectively in models that included both MAT and MAP; both climate metrics were significant and shared little explanatory power. Table 2 Multiple regression analyses of live fine-root stoichiometry. Full size table Climate data (MAT and MAP) collectively explained 7–34% of the variation in fine-root C, N, P and stoichiometric ratios ( Table 2 ). Available soil N and P data explained between 43–75% of the variation in fine-root C, N, P and stoichiometric ratios; however, only a small fraction of all fine-root data had associated soil data. When soil N and P data were also taken into account, the climate variables accounted for a partial 16–22% of the variation in N, P and stoichiometric ratios, less than they explained on their own because of the correlation between climate variables and soil nutrients at the global scale. Climatic data (MAT and MAP) combined with soil data (N and P contents) explained surprisingly high proportions of root nutrient variation: 59, 76 and 73% of the global variation in fine-root N, P and N:P, respectively ( Table 2 ). Allometric scaling of N and P When all data were pooled, live fine-root N and P were correlated with a standardized major axis (SMA) log-log slope of 0.764, which was slightly greater than that of green leaves (SMA log-log slope=0.676) ( Fig. 3 ). The variation in fine-root N and P across all biomes shared much of the trait space found in the global data sets of green-leaf nutrient concentrations ( Fig. 3 ). However, average concentrations of both N and P in fine roots (10.2 mg g −1 N and 0.83 mg g −1 P) were lower than those in green leaves (20.1 mg g −1 N and 1.77 mg g −1 P). Differences in slopes and intercepts of the N versus P relations result in leaves having higher N on average than roots at any common P level. 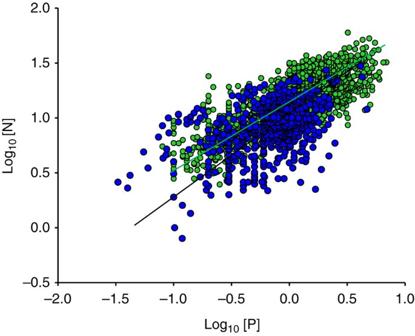Figure 3: Allometric scaling of N and P in fine roots and green leaves. Blue and green circles indicate fine roots and green leaves, respectively. The N and P concentration values (mg g−1) were log-transformed (base 10). The relationships between N and P in fine roots and green leaves are best described by a linear function-based SMA (fine roots: log10N=1.045+0.764×log10P,n=731,r2=0.232, 95% C.I. for slope=0.717–0.813,P<0.001, blue circles with blue trend line; green leaves: log10N=0.629×log10P+1.192,n=2287,r2=0.505, 95% C.I. for slope=0.617–0.642,P<0.001, green circles with green trend line). Global data sets for green leaves from references6,15,42. Figure 3: Allometric scaling of N and P in fine roots and green leaves. Blue and green circles indicate fine roots and green leaves, respectively. The N and P concentration values (mg g −1 ) were log-transformed (base 10). The relationships between N and P in fine roots and green leaves are best described by a linear function-based SMA (fine roots: log 10 N=1.045+0.764×log 10 P, n =731, r 2 =0.232, 95% C.I. for slope=0.717–0.813, P <0.001, blue circles with blue trend line; green leaves: log 10 N=0.629×log 10 P+1.192, n =2287, r 2 =0.505, 95% C.I. for slope=0.617–0.642, P <0.001, green circles with green trend line). Global data sets for green leaves from references [6] , [15] , [42] . Full size image The higher N:P ratio in less nutrient-rich coarse roots than in fine roots indicates that P concentration decreases proportionally more than N concentration with increasing root size. This could be a result of more translocation of P than N from coarse to fine roots or more likely reflect different proportional allocation of C, N and P to new biomass as roots grow from very fine to fine to coarse root status. Regardless of the mechanism, the differences in N:P ratio with root size support the idea of reduced P requirements for old and slow-growing coarse roots [26] . Overall, these results provide support for the growth rate hypothesis [25] , [27] that predicts faster growing tissues such as fine roots rather than coarse roots need relatively more P-rich RNA to support rapid protein synthesis and thus exhibit lower tissue N:P and C:P ratios. Despite the importance to plant nutrition of nutrient retranslocation from senescing leaves, knowledge of whether similar processes occur in senescing roots is still remarkably limited [26] , [28] . Based on our compiled data, when N and P concentrations in live and dead roots are compared ( Table 1 ), there was no evidence for N retranslocation but there was evidence of P retranslocation (averaging 27% overall). These results were virtually identical if limited to samples with both live and dead root elemental measurements. Evidence for P retranslocation conflicts with the single most cited study investigating whether nutrients are retranslocated from fine roots [28] , which found no evidence of retranslocation for N, P, K or Mg in a single pine species ( Pinus radiata ), but is consistent with a similar analysis based on data synthesis [26] . Note that there are enormous methodological challenges to quantifying retranslocation in roots, compared with leaves [26] . Clearly, important advances in this area remain to be made. Compared with previous root studies, the average C:N:P in live roots of 2≤Φ<5 mm in diameter (1,078:16:1) was similar to those reported by Gordon & Jackson [26] (920:12:1). The average C:N:P in live fine roots (906:15:1), however, differs from previous results reported by Jackson et al . [1] (450:11:1) and by Gordon & Jackson [26] (522:12:1). This difference is likely a result of different sample sizes, that is, 258 versus 13 for C, 1,003 versus 54 for N and 534 versus 41 for P in this study versus Jackson et al . [1] and Gordon & Jackson [26] . A larger proportion of fine-root data (74%) from larger live fine roots (1≤Φ<2 mm diameter) probably also contributed to higher C:N:P in this study. The C:N:P and N:P ratios in live roots (1,053:16:1) was similar to those reported for green leaves (N:P of 13.8 by Reich and Oleksyn [6] , P= 0.271; 18.2 by Wright et al . [15] , P= 0.120; one-way ANOVA; C:N:P of 1,212:16:1 (refs 8 , 29 , 30 )), indicating that live plant tissues from terrestrial ecosystems share a common functional stoichiometry. Also similar to that in senesced leaves (1,016:19:1) [9] , the C:N:P ratio was 1,059:20:1 for all sized dead roots and 844:19:1 for dead fine roots, suggesting that terrestrial C:N:P ratios, both in leaves and roots, are equally well constrained at the level of ecosystems as are marine ratios [27] . The exponential and linear declines with latitude in live roots and green leaves, respectively, imply some similar and different mechanisms for latitudinal N:P variations in roots versus leaves. The latitudinal gradient in soil N versus P availability across latitudes [14] , [21] (soil N is less limited than P across many low-latitude tropical forests [31] ) could explain the latitudinal N:P declines in both leaves and roots. As fine-root P increased positively, but fine-root N remained relatively constant with latitude ( Table 2 ), the fine-root N:P ratio declined exponentially, as N:P is an inverse function of latitude. By contrast, the increased green-leaf P with latitudes is accompanied by a increased green-leaf N [6] ; consequently, the N:P decline with increasing latitude in green leaves is not as abrupt as in roots. However, the underlying mechanisms for the differences in the latitudinal N patterns between the fine roots and green leaves are not clear. McGroddy et al . [8] proposed that the exceptional ability to resorb P in P-poor conditions, but constrained ability to resorb N in N-poor conditions (owing to the tendency for plants to use some N in proteins that are structural and/or difficult to resorb) could contribute to the differences in N:P trends between the linear decline in green leaves and the exponential decline in litterfall [8] , [32] . A similar difference in live and dead root biogeography would require both that roots routinely resorb nutrients prior to senescence and that resorption of P is stronger than of N in P-poor conditions. Our results, however, show exponential N:P declines with latitude both in live and dead roots ( Fig. 1 ). The data in our compilation suggests that there is apparently no N resorption but considerable P resorption in fine roots (27%, Table 1 ), supporting the idea that P can be resorbed more easily than N [8] ; but this resorption pattern shows no latitudinal trend (as evidenced by the parallel variation in live and dead N:P). Because the samples from the field include both functionally active (live) and inactive (dead) roots, which are not often separated in some original studies owing to the difficulty in distinguishing them, the observed exponential trends in roots do not clearly answer whether the proposed mechanism for leaves [8] may also be applicable to root systems. Moreover, roots also differ significantly from leaves (such as lack of morphologically distinct abscission zones and still closely associating with soils after death) that will influence the nutrient resorption and contents in root systems. Further studies will be required before firm conclusions can be made about similarities or differences in biogeographical variation in live versus senesced root and leaf chemistry. The differences in fine-root N, P and N:P ratio among biomes, with high N:P ratios both in roots ( Fig. 2 ) and in leaves [6] , [8] , [9] , [15] in tropics, support the idea that variations in P rather than N regulates the large-scale cross-continental biogeochemical patterns of plant N:P stoichiometry and nutrient use strategies [4] , [14] , [21] . The findings of fine-root C, N, P and their ratios in relation to climatic variable and soil variables ( Table 2 ) also again confirmed the latitudinal N:P decline patterns in fine roots ( Fig. 1 ). The analyses for soil N and P ( Table 2 ) were based on a much smaller data set than relations with climate metrics. In a model with all four soil and climate parameters, the fine-root P and N:P ratios were related to soil P and to all climatic variables, especially to MAP, likely reflecting the close correlation between soil P and MAP which results from the occurrence of poor leached soils in tropical areas with high precipitation [14] . The significant correlations between fine-root N:P and soil P, together with the observed root ( Fig. 1 ) and leaf latitudinal N:P patterns [6] , [8] , appear to support the geochemical hypothesis [11] , [14] , [20] , that is, tropical soils are on average geologically older, more weathered with lower supply of P relative to N, consequently resulting in higher N:P ratios in roots in tropical latitudes. The variation not explained by climate and soil ( Table 2 ) is likely in part due to biological factors, for example, plant species (such as differences in nutrient economy), stand age and disturbance history [12] , [33] . Differences in slopes and intercepts of the N versus P relations result in leaves having higher N on average than roots at any common P level ( Fig. 3 ). One possible explanation for this difference involves the greater requirement for N in leaves because of the need for N-rich Rubisco in leaves. Leaves and roots differ in respiratory carbon-to-nitrogen relations, likely for this reason [17] , suggesting that it may also be involved in N:P differences among leaves and roots. In summary, despite the variability in biomes, species and soil types, our analyses indicate the existence of global patterns in fine-root N, P and N:P ratio along latitudinal gradients, adding support to a widely held belief in ecosystem ecology that plants in tropical habitats are generally more P-limited than those at higher latitudes [14] . These biogeographic gradients exist likely as a result of the collective influences of complex interactions of climate, soil and biological factors that change in relation to the distance from the equator. Differences in N:P ratios were largely due to variation in root P and were associated with variation in soil P rather than soil N, supporting the hypothesis that global latitudinal patterns of plant N:P are driven largely by soil P. The decline of fine-root N:P with latitude and the allometric scaling of fine-root N versus P also provide support for the latitudinal compensation hypothesis [22] , [23] , [24] and the growth rate hypothesis [25] ,which predicts that selection for rapid-growth with short-growth seasons in high latitudes increases tissue P-content disproportionately (and thus a lower N:P). As the growth rate hypothesis [25] predicts, the biota can modify the strength of the geochemical influence through plant-soil feedbacks to the N and P cycles, leading to coupling between climate, ecological process and resultant stoichiometric patterns [20] , [34] . Data compilation We collected data on C, N and P in roots from a range of literature sources ( Supplementary References ). The extensive literature search through five databases: ISI Web of Science, PubMed, Google Scholar, JSTOR and Scirus, was conducted using keywords of 'fine root*' and 'nutrient*'. We did not include data from either fertilized experiments in natural environments or the experiments conducted in pots or greenhouses. We included data that had measured roots to at least 20 cm depth in the soil. The data were averaged for the particular site, if studies provided data for multiple times and locations within a site. We used the Global Gazetteer Version 2.2 ( http://www.fallingrain.com/world/ ) to determine the latitude, longitude or altitude if this information was missing in the original paper. Soil total N and P data were from the original papers or other studies that were conducted in the same sites. Our data cover a wide range of ecosystems, including arctic tundra, forests, grasslands, wetlands and deserts. We further classified forests into three biomes: boreal, temperate and tropical. Boreal forests included all forests occurring between 46°N and 66°N latitude [35] , tropical forests included all forests occurring between 23.5°S and 23.5°N latitude [36] , and temperate forests included all forests between the tropical and boreal latitudes. Study sites varied in stand ages and included both natural and manipulated ecosystems. The total data set represented 527 sites, including 40 sites subjected to recent disturbances (stand age <20 years). Site elevation ranges from 3 to 3,520 m. MAT ranges from −9 to 30 °C; mean annual rainfall ranges from 170 to 10,370 mm per year.. Statistical analysis Means of root N and P and their ratios were compared among root size classes (Φ<1, 1≤Φ<2, 2≤Φ<5 and Φ≥5 mm) by using one-way analysis of variance, followed by Tukey's post hoc comparisons when effects were significant. Because of the limited number of samples, dead roots were pooled for all size classes. The overall means in Table 1 are based on all observations (thus weight size classes by their sampling intensity) and the ratio columns, by default, include only samples with both elements measured, whereas the C, N and P columns include all observations. Weighting overall means equally by all size classes and comparing element means only for those with multiple values per sample does modify the absolute values but does not change the patterns or conclusions of the study. The relationships between N:P ratios in roots of all diameter classes and latitude were fitted by power functions. Because of the limited number of samples available for roots ≥2 mm in diameter ( Table 1 ), further analysis was conducted only for fine roots (<2 mm in diameter). Fine-root N:P, C:N and C:P ratios were transformed using base-10 logarithm in order to meet the assumptions of normality and homogeneity of variances. The log transformation eliminated any major departures from normality or homogeneity of variances, as is commonly used in analyses of leaf and root traits [9] , [17] , [37] . Multiple regression analysis with backward stepwise procedure was used to examine the overall patterns of response of fine-root N and P and their ratios to climatic (MAT and precipitation) and soil variables. Regression models were developed with increasing numbers of independent variables. The models labelled 'Climate+Soil' include MAT, MAP, soil N and P as explanatory variables ( Table 2 ). Overall model significance and goodness-of-fit were judged by using the likelihood ratio statistic and assessing change in Akaike's information criterion scores. A substantial change is considered when a change in Akaike's information criterion of >2 in the descriptive ability of the final model over the alternatives [38] . To describe joint variation of N and P concentrations in both fine roots and green leaves, we used SMA regression, a Model II regression method recommended when the variables can not be clearly separated into independent or dependent, and when error is associated with the measures of both [39] . After fine-root and green-leaf nutrient concentration values (mg g −1 ) were log-transformed (base 10), the Model II regression analysis was performed in R by using the SMATR package (version 2.1) [40] . Two-tailed t -tests were used to determine whether the slopes were significantly different. All statistical analyses were performed in R for Window version 2.10.1 statistical software [41] . Data sets for green leaves were pooled from Reich & Oleksyn [6] , Wright et al . [15] , Townsend et al . [42] , and for senesced leaves, from McGroddy et al . [8] and Yuan & Chen [9] . Data references for dead roots are indicated by a star in the Supplementary References . How to cite this article: Yuan, Z. Y. et al . Global-scale latitudinal patterns of plant fine-root nitrogen and phosphorus. Nat. Commun. 2:344 doi: 10.1038/ncomms1346 (2011).